Experimental simulation of closed timelike curves Closed timelike curves are among the most controversial features of modern physics. As legitimate solutions to Einstein’s field equations, they allow for time travel, which instinctively seems paradoxical. However, in the quantum regime these paradoxes can be resolved, leaving closed timelike curves consistent with relativity. The study of these systems therefore provides valuable insight into nonlinearities and the emergence of causal structures in quantum mechanics—essential for any formulation of a quantum theory of gravity. Here we experimentally simulate the nonlinear behaviour of a qubit interacting unitarily with an older version of itself, addressing some of the fascinating effects that arise in systems traversing a closed timelike curve. These include perfect discrimination of non-orthogonal states and, most intriguingly, the ability to distinguish nominally equivalent ways of preparing pure quantum states. Finally, we examine the dependence of these effects on the initial qubit state, the form of the unitary interaction and the influence of decoherence. One aspect of general relativity that has long intrigued physicists is the relative ease with which one can find solutions to Einstein’s field equations that contain closed timelike curves (CTCs)—causal loops in space–time that return to the same point in space and time [1] , [2] , [3] . Driven by apparent inconsistencies—like the grandfather paradox—there have been numerous efforts, such as Novikov’s self-consistency principle [4] to reconcile them or Hawking’s chronology protection conjecture [5] , to disprove the existence of CTCs. While none of these classical hypotheses could be verified so far, the situation is particularly interesting in the quantum realm. In his seminal 1991 paper Deutsch [6] showed for quantum systems traversing CTCs that there always exist unique solutions, which do not allow superluminal signalling [7] . Quantum mechanics therefore allows for causality violation without paradoxes, while remaining consistent with relativity. Advances in the field of Deutsch CTCs have shown some very surprising and counter-intuitive results, such as the solution of NP-complete problems in polynomial time [8] , unambiguous discrimination of any set of non-orthogonal states [9] , perfect universal quantum state cloning [10] , [11] and the violation of Heisenberg’s uncertainty principle [12] . The extraordinary claims of what one could achieve given access to a quantum system traversing a CTC have been disputed in the literature, with critics pointing out apparent inconsistencies in the theory, such as the information paradox or the linearity trap [13] , [14] . However, it has been shown that the theory can be formulated in such a way that these inconsistencies are resolved [7] , [15] . Modern experimental quantum simulation allows one to ask meaningful questions that provide insights into the behaviour of complex quantum systems. Initial results have been obtained in various areas of quantum mechanics [16] , [17] , [18] and in particular in the field of relativistic quantum information [19] , [20] , [21] , [22] , [23] . This recent experimental success, coupled with the growing interest in the study of nonlinear extensions to quantum mechanics, motivates the question of whether the fundamentally nonlinear dynamics and the unique behaviour arising from CTCs can be simulated experimentally. In this article we use photonic systems to simulate the quantum evolution through a Deutsch CTC. We demonstrate how the CTC-traversing qubit adapts to changes in the input state | ψ 〉, and unitary interaction U to ensure physical consistency according to Deutsch’s consistency relation [6] . We observe nonlinear evolution in the circuit suggested by Bacon [8] and enhanced distinguishability of two non-orthogonal states after the action of an optimized version of a circuit proposed by Brun et al. [9] Using the self-consistent formulation of ref. 7 we then move beyond the simplest implementations and find a striking difference in the behaviour of the system for direct as opposed to entanglement-assisted state preparation. Finally, we explore the system’s sensitivity to decoherence. The Deutsch model While there has been some recent success on alternative models of CTCs based on post-selection [23] , [24] , [25] , we focus on the most prominent model for describing quantum mechanics in the presence of CTCs, introduced by Deutsch [6] . Here a quantum state | ψ 〉 interacts unitarily with an older version of itself ( Fig. 1 ). With the inclusion of an additional swap gate, this can equivalently be treated as a two-qubit system, where a chronology-respecting qubit interacts with a qubit ρ CTC trapped in a CTC. 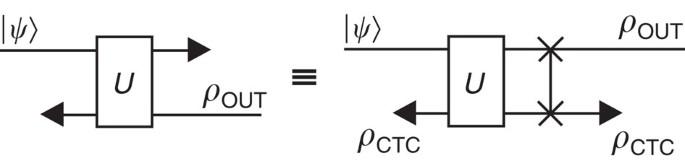Figure 1: Model of a quantum state |ψ〉interacting with an older version of itself. This situation can equivalently be interpreted as a chronology-respecting qubit interacting with a qubit trapped in a CTC. The CTC in general consists of a causal worldline with its past and future ends connected via a wormhole (indicated by black triangles). The quantum state of ρ CTC in this picture is determined by Deutsch’s consistency relation: Figure 1: Model of a quantum state | ψ 〉 interacting with an older version of itself. This situation can equivalently be interpreted as a chronology-respecting qubit interacting with a qubit trapped in a CTC. The CTC in general consists of a causal worldline with its past and future ends connected via a wormhole (indicated by black triangles). Full size image where U ′ is the unitary U followed by a SWAP gate ( Fig. 1 ). This condition ensures physical consistency—in the sense that the quantum state may not change inside the wormhole—and gives rise to the nonlinear evolution of the quantum state | ψ 〉. The state after this evolution is consequently given by ρ OUT =Tr 2 [ U ′(| ψ 〉〈 ψ | ⊗ ρ CTC ) U ′ † ]. The illustration in Fig. 1 further shows that the requirement of physical consistency forces ρ CTC to adapt to any changes in the surroundings, such as a different interaction unitary U or input state | ψ 〉. While equation (1) is formulated in terms of a pure input state | ψ 〉, it can be directly generalized to mixed inputs [7] . Simulating CTCs Our experimental simulation of a qubit in the (pure) state | ψ 〉 traversing a CTC relies on the circuit diagram shown in Fig. 2a ). A combination of single-qubit unitary gates before and after a controlled-Z gate allows for the implementation of a large set of controlled-unitary gates U . Using polarization-encoded single photons, arbitrary single-qubit unitaries can be realized using a combination of quarter-wave (QWP) and half-wave plates (HWP); additional SWAP gates before or after U are implemented as a physical mode swap. The controlled-Z gate is based on non-classical (Hong-Ou-Mandel) interference of two single photons at a single partially polarizing beam splitter (PPBS) that has different transmittivities η V =1/3 for vertical (V) and η H =1 for horizontal (H) polarization [26] —a more detailed description of the implementation of the gate can be found in ref. 27 . Conditioned on post-selection, it induces a π phase shift when the two interfering single-photon modes are vertically polarized, such that | VV 〉→−| VV 〉 with respect to all other input states. 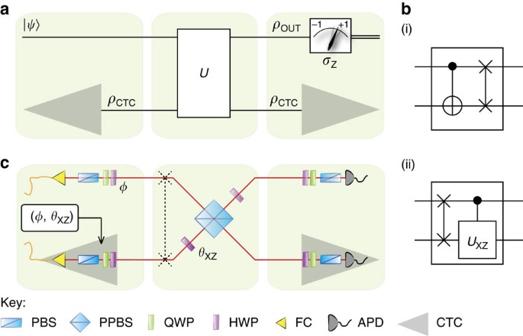Figure 2: Experimental details. (a) The circuit diagram for a general unitary interactionUbetween the state |ψ〉 and the CTC system. (b) The specific choice of unitary in the demonstration of the (i) nonlinear evolution and (ii) perfect discrimination of non-orthogonal states. (c) Experimental setup for case (ii). Two single photons, generated via spontaneous parametric down-conversion in a nonlinear β-barium-borate crystal, are coupled into two optical fibres (FC) and injected into the optical circuit. Arbitrary polarization states are prepared using a Glan–Taylor polarizer (POL), a quarter-wave (QWP) and a half-wave plate (HWP). Non-classical interference occurs at the central partially polarizing beam splitter (PPBS) with reflectivitiesηH=0 andηV=2/3. Two avalanche photo-diodes (APDs) detect the single photons at the outputs. The states |Ψ〉 are chosen in thex–zplane of the Bloch sphere, parameterized byϕ, and CUxzis the corresponding controlled unitary, characterized by the angleθxz. TheSWAPgate was realized via relabelling of the input modes. Figure 2: Experimental details. ( a ) The circuit diagram for a general unitary interaction U between the state | ψ 〉 and the CTC system. ( b ) The specific choice of unitary in the demonstration of the (i) nonlinear evolution and (ii) perfect discrimination of non-orthogonal states. ( c ) Experimental setup for case (ii). Two single photons, generated via spontaneous parametric down-conversion in a nonlinear β-barium-borate crystal, are coupled into two optical fibres (FC) and injected into the optical circuit. Arbitrary polarization states are prepared using a Glan–Taylor polarizer (POL), a quarter-wave (QWP) and a half-wave plate (HWP). Non-classical interference occurs at the central partially polarizing beam splitter (PPBS) with reflectivities η H =0 and η V =2/3. Two avalanche photo-diodes (APDs) detect the single photons at the outputs. The states | Ψ 〉 are chosen in the x–z plane of the Bloch sphere, parameterized by ϕ , and CU xz is the corresponding controlled unitary, characterized by the angle θ xz . The SWAP gate was realized via relabelling of the input modes. Full size image One of the key features of a CTC is the inherently nonlinear evolution that a quantum state | ψ 〉 undergoes when traversing it. This is a result of Deutsch’s consistency relation, which makes ρ CTC dependent on the input state | ψ 〉. In order to simulate this nonlinear behavior using linear quantum mechanics we make use of the effective nonlinearity obtained from feeding extra information into the system. In our case we use the classical information about the preparation of the state | ψ 〉 and the unitary U to prepare the CTC qubit in the appropriate state ρ CTC as required by the consistency relation equation (1). After the evolution we perform full quantum state tomography on the CTC qubit in order to verify that the consistency relation is satisfied. Nonlinear evolution As a first experiment we investigate the nonlinearity by considering a Deutsch CTC with a CNOT interaction followed by a SWAP gate as illustrated in Fig. 2b(i) . This circuit is well known for the specific form of nonlinear evolution: which has been shown to have important implications for complexity theory, allowing for the solution of NP-complete problems with polynomial resources [8] . According to Deutsch’s consistency relation (equation (1)) the state of the CTC qubit for this interaction is given by We investigate the nonlinear behaviour experimentally for 14 different quantum states , with and a variety of phases φ ∈ {0, 2 π }, where the locally available information ϕ and φ is used to prepare ρ CTC . In standard (linear) quantum mechanics no unitary evolution can introduce additional distinguishability between quantum states. To illustrate the nonlinearity in the system we thus employ two different distinguishability measures: the trace distance , where , and a single projective measurement with outcomes ‘+’ and ‘−’: While the metric is a commonly used distance measure, it does not have an operational interpretation and requires full quantum state tomography in order to be calculated experimentally. The measure in contrast is easily understood as the probability of obtaining different outcomes in minimum-error discrimination of the two states using a single projective measurement on each system. The operational interpretation and significance of is discussed in more detail in the Supplementary Note 1 . Both and are calculated between the state | ψ 〉 and the fixed reference state | H 〉 after being evolved through the circuit shown in Fig. 2b(i) . The results are plotted and compared to standard quantum mechanics in Fig. 3 . If the state | ψ 〉 is not known then, based only on the knowledge of the reference state | H 〉 and the evolution in equation (2) it is natural and optimal to use the measure with a σ z -measurement. 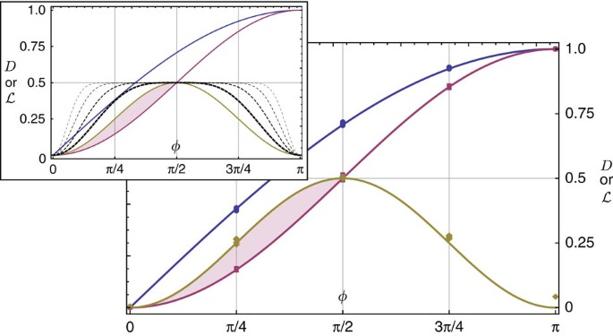Figure 3: Nonlinear evolution in a Deutsch CTC withSWAP.CNOTinteraction. Both the trace distance and theσz-based distinguishability measure (equal to within experimental error in this case) of the evolved statesρOUTafter the interaction with the CTC are shown as yellow diamonds. The blue circles (red squares) represent the measure () between the input states |ψ〉 and |H〉 in the case of standard quantum mechanics. Note that due to the phase independence of the evolution in equation (2), states that only differ by a phase collapse to a single data point. Crucially, the metric does not capture the effect of the nonlinearity, while does, indicated by the red-shaded region. Error bars obtained from a Monte Carlo routine simulating the Poissonian counting statistics are too small to be visible on the scale of this plot. Inset: The dashed black lines with decreasing thickness represent theoretical expectations for and from 2, 3, 4 and 5 iterations of the circuit. Figure 3: Nonlinear evolution in a Deutsch CTC with SWAP.CNOT interaction. Both the trace distance and the σ z -based distinguishability measure (equal to within experimental error in this case) of the evolved states ρ OUT after the interaction with the CTC are shown as yellow diamonds. The blue circles (red squares) represent the measure () between the input states | ψ 〉 and | H 〉 in the case of standard quantum mechanics. Note that due to the phase independence of the evolution in equation (2), states that only differ by a phase collapse to a single data point. Crucially, the metric does not capture the effect of the nonlinearity, while does, indicated by the red-shaded region. Error bars obtained from a Monte Carlo routine simulating the Poissonian counting statistics are too small to be visible on the scale of this plot. Inset: The dashed black lines with decreasing thickness represent theoretical expectations for and from 2, 3, 4 and 5 iterations of the circuit. Full size image We observe enhanced distinguishability for all states with an initial trace distance to | H 〉 smaller than (that is, ), as clearly demonstrated by the σ z -based measure, see Fig. 3 . Note, however, that this advantage over standard quantum mechanics is not captured by the metric ( ρ 1 , ρ 2 ) unless the nonlinearity is amplified by iterating the circuit on the respective output at least three times, see the inset of Fig. 3 . This shows that the nonlinearity is not directly related to the distance between two quantum states. By testing states with various polar angles for each azimuthal angle on the Bloch sphere, we confirm that any phase information is erased during the evolution and that the evolved state ρ OUT is indeed independent of φ , up to experimental error. We further confirm, with an average quantum state fidelity of F =0.998(2) between the input and output states of ρ CTC in equation (3), that the consistency relation (1) is satisfied for all tested scenarios. Non-orthogonal state discrimination While it is the crucial feature, nonlinear state evolution is not unique to the SWAP.CNOT interaction, but rather a central property of all non-trivial CTC interactions. Similar circuits have been found to allow for perfect distinguishability of non-orthogonal quantum states [9] , leading to discomforting possibilities such as breaking of quantum cryptography [9] , perfect cloning of quantum states [10] , [11] and violation of Heisenberg’s uncertainty principle [12] . In particular it has been shown that a set of N distinct quantum states in a space of dimension N can be perfectly distinguished using an N -dimensional CTC system. The algorithm proposed by Brun et al. [9] relies on an initial SWAP operation between the input and the CTC system, followed by a series of controlled unitary operations, transforming the input states to an orthogonal set, which can then be distinguished. In our simulation of this effect we consider the qubit case N =2, which consequently would require two controlled unitary operations between the input state and the CTC system. We note, however, that without loss of generality the set of states to be discriminated can be rotated to the x–z plane of the Bloch sphere, such that | ψ 0 〉=| H 〉 and for some angle ϕ . In this case, the first controlled unitary is the identity operation , while the second performs a controlled rotation of | ψ 1 〉 to | V 〉 as illustrated in Fig. 4a ). In detail, the gate CU xz applies a π rotation to the target qubit conditional on the state of the control qubit, about an axis in the x–z plane defined by the angle θ xz . For the optimal choice the gate rotates the state | ψ 1 〉 to | V 〉, orthogonal to | ψ 0 〉, enabling perfect distinguishability by means of a projective σ z measurement (see Fig. 4a ). 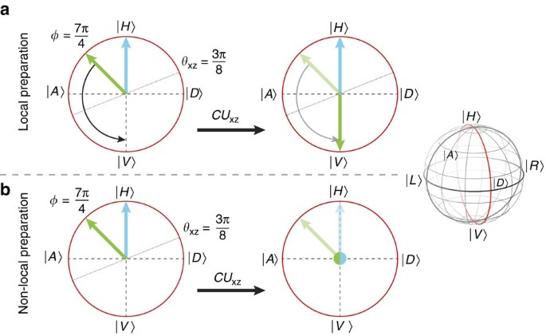Figure 4: Bloch-sphere evolution of states traversing a CTC. In the case of (a) local state preparation, the state |ψ0〉=|H〉 (blue) is unaffected by CUxz, while |Ψ1〉 (green) undergoes aπrotation about the axis defined byθxz. The axis is chosen assuch that, which can then be perfectly distinguished from |ψ0〉. (b) For non-local preparation of the initial states and the same choice ofθxzthe controlled unitary maps both initial states to the maximally mixed state. The probability of distinguishing the two states is therefore 1/2—as good as randomly guessing. Figure 4: Bloch-sphere evolution of states traversing a CTC. In the case of ( a ) local state preparation, the state | ψ 0 〉=| H 〉 (blue) is unaffected by CU xz , while | Ψ 1 〉 (green) undergoes a π rotation about the axis defined by θ xz . The axis is chosen as such that , which can then be perfectly distinguished from | ψ 0 〉. ( b ) For non-local preparation of the initial states and the same choice of θ xz the controlled unitary maps both initial states to the maximally mixed state . The probability of distinguishing the two states is therefore 1/2—as good as randomly guessing. Full size image In practice the gate CU xz is decomposed into a controlled-Z gate between appropriate single-qubit rotations, defining the axis θ xz . The latter are realized by half-wave plates before and after the PPBS, set to an angle of θ xz /4 with respect to their optic axis (see Fig. 2c ): Note that relation (1) requires that ρ CTC =| H 〉〈 H |, whenever the input state is | H 〉, independent of the gate CU xz . Crucially, this consistency relation ensures that any physical CTC system adapts to changes in ϕ and θ xz , parameterizing the input state and gate, respectively. In our simulation these two parameters are used to prepare the corresponding state ρ CTC , as shown in Fig. 2c . In a valid experimental simulation the input and output states ρ CTC have to match, that is, ρ CTC has to satisfy relation (1). This has been verified for all following experiments with an average quantum state fidelity of =0.996(7). In the experiment, we prepared near-pure quantum states directly on single photons using a Glan–Taylor polarizer followed by a combination of a HWP and a QWP. We simulated CTC-aided perfect discrimination of non-orthogonal states for 32 distinct quantum states | ψ 1 〉 with ϕ ∈ [0, 2 π ). For each state we implemented CU xz with the optimal choice of . Furthermore, we tested the ability of this system to distinguish the set {| ψ 0 〉, | ψ 1 〉} given non-optimal combinations of ϕ and θ xz . For this we either chose ϕ =3 π /2 and varied the gate over the full range of , or chose CU xz as a controlled Hadamard (optimal for ϕ =3 π /2) and varied the state | ψ 1 〉 over the full range of ϕ ∈ [0, 2 π ). The output state is characterized by quantum state tomography, which provides sufficient data to obtain for arbitrary measurement directions as well as for the calculation of the trace distance. 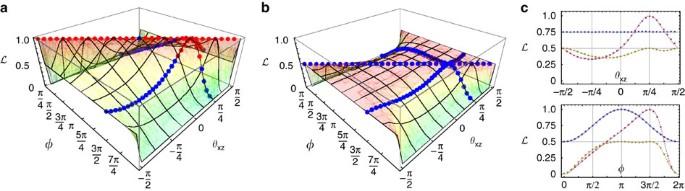Figure 5: Experimental results. Probability of state discrimination for (a) locally prepared and (b) non-locally prepared states |ψ0〉=|H〉 andas measured by . The surface represents the theoretically predicted probability depending on the state and gate parametersϕandθxz, respectively. Solid, red (open, blue) data points indicate better (worse) performance than standard quantum mechanics. (c) Cross-sectional views of the combined plotsaandbreveal the rich structure in the dependencies on the initial parameters for (top) a fixed state (ϕ=3π/2) and (bottom) a fixed gate (θxz=π/4). Here red squares (yellow diamonds) correspond to the CTC case with local (non-local) preparation and blue circles represent standard quantum mechanics. Error bars obtained from a Monte Carlo routine simulating the Poissonian counting statistics are too small to be visible on the scale of this plot. Figure 5a illustrates the observed distinguishability for the above experiments and compares it to the expectation from standard quantum mechanics. In the latter case the measure is maximized by choosing the optimal projective measurement, based on the available information about the states | ψ 0 〉 and | ψ 1 〉. Crucially, the optimized L is directly related to the trace distance as and therefore captures the same qualitative picture, without the requirement for full quantum state tomography. In the CTC case a σ z -measurement is chosen, which is optimal when . Otherwise further optimization is possible based on the knowledge of θ xz (see Supplementary Note 2 and Supplementary Fig. 1 for more details). Furthermore, we note that the above scenario can also be interpreted in a state-identification rather than state-discrimination picture, which is discussed in more detail in Supplementary Note 3 and Supplementary Fig. 2 . Figure 5: Experimental results. Probability of state discrimination for ( a ) locally prepared and ( b ) non-locally prepared states | ψ 0 〉=| H 〉 and as measured by . The surface represents the theoretically predicted probability depending on the state and gate parameters ϕ and θ xz , respectively. Solid, red (open, blue) data points indicate better (worse) performance than standard quantum mechanics. ( c ) Cross-sectional views of the combined plots a and b reveal the rich structure in the dependencies on the initial parameters for (top) a fixed state ( ϕ =3 π /2) and (bottom) a fixed gate ( θ xz = π /4). Here red squares (yellow diamonds) correspond to the CTC case with local (non-local) preparation and blue circles represent standard quantum mechanics. Error bars obtained from a Monte Carlo routine simulating the Poissonian counting statistics are too small to be visible on the scale of this plot. Full size image Local versus non-local state preparation Owing to the inherent nonlinearity in our simulated system, care must be taken when describing mixed input states ρ in . In particular a distinction between proper and improper mixtures can arise, which is unobservable in standard (linear) quantum mechanics [28] . This ambiguity is resolved in ref. 7 by requiring the consistency condition to act shot-by-shot—that is, independently in every run of the experiment—on the reduced density operator of the input state. For proper mixtures this means that ρ in is always taken as a pure state, albeit a different one shot-by-shot. For improper mixtures in contrast, ρ in will always be mixed. A similar, but much more subtle and fascinating feature that has received less attention in the literature so far occurs with respect to preparation of pure states [29] . While in standard quantum mechanics a pure state prepared directly (locally) on a single qubit is equivalent to one that has been prepared non-locally through space-like separated post-selection of an entangled resource state, this is not true under the influence of a CTC. The origin of this effect is not the nonlinear evolution, but rather the local absence of classical information about the post-selection outcome. The role of locally available classical information in entanglement-based preparation schemes is a matter of current debate and still to be clarified. A possible resource state for alternatively preparing | ψ 0 〉 and | ψ 1 〉 could be of the form , where projection of the first qubit onto the state |0〉 and |1〉 leaves the second qubit in the state | ψ 0 〉 and | ψ 1 〉, respectively. From the point of view of ρ CTC , however, there exists no information about the outcome of this projective measurement. Hence it ‘sees’ and adapts to the mixed state . The state of the CTC qubit is therefore different for local and non-local preparation. If this was not the case, it would enable superluminal signalling, which is in conflict with relativity [29] . Figure 4b ) illustrates the evolution induced by CU xz , when the input states | H 〉 and | ψ 1 〉 are prepared using an entangled resource |Ψ〉, rather than directly. The results of the previously discussed distinguishability experiments for this case are shown in Fig. 5b ). In Fig. 5c ) they are compared to the case of local preparation and to standard quantum mechanics for a fixed input state and a fixed gate, respectively. Again, consistency of our simulation is ensured by a quantum state fidelity of =0.9996(3) between the input and output states of ρ CTC . In our simulation we find that the CTC system can indeed achieve perfect distinguishability of the (directly prepared) states | ψ 0 〉 and | ψ 1 〉 even for arbitrarily close states if the appropriate gate is implemented (see Fig. 5a ). Furthermore, we show that the advantage over standard quantum mechanics persists for a wide range of non-optimal gate–state combinations, outside of which, however, the CTC system performs worse (blue points). Notably, we find that for non-locally prepared input states CTC-assisted state discrimination never performs better than random guessing—a probability of (as shown in Fig. 5b ). The predictions for standard quantum mechanics, in contrast are independent of the way the states | ψ 0 〉 and | ψ 1 〉 are prepared. Decoherence We further investigated the effect of two important decoherence mechanisms on the simulated CTC system (shown in Fig. 2a ). The first is a single-qubit depolarizing channel acting on the input state | ψ 〉, which can be modelled as where ( σ x , σ y , σ z ) are the three Pauli matrices and p ∈ [0, 1] quantifies the amount of decoherence. The second form of decoherence concerns the controlled unitary CU xz and is described as where ε ∈ [0, 1] is the probability of the gate to fail, describing the amount of decoherence that is present. For ε =0 the gate acts as an ideal controlled rotation CU xz , while it performs the identity operation for ε =1. We tested the robustness of the state-discrimination circuit in Fig. 2b (ii) against both forms of decoherence. For this test we chose CU xz as a controlled Hadamard (that is, θ xz = π /4) and the initial states | ψ 0 〉=| H 〉 and (that is, ϕ =3 π /2). Fig. 6 shows the distinguishability of the evolved states as a function of both decoherence mechanisms over the whole range of parameters p ∈ [0, 1] and ε ∈ [0, 1]. Note that the decoherence channel in equation (7) does not have an analogue in the standard quantum mechanics case (that is, without a CTC); hence only the channel in equation (6) is considered for comparison. It is further naturally assumed that the experimenter has no knowledge of the specific details of the decoherence and therefore implements the optimal measurements for the decoherence-free case. The physical validity of the simulation is ensured by the consistency of ρ CTC across the boundary of the wormhole with an average fidelity of =0.997(4). 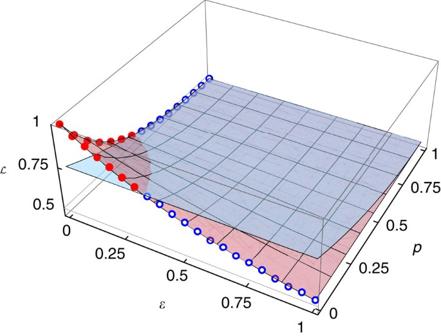Figure 6: State discrimination as a function of gate and qubit decoherence for locally prepared states. Hereεquantifies the decoherence of the unitary interaction CUxz(withθxz=π/4), which has no analogue in the standard quantum mechanics case, andpthe single-qubit depolarization of the input qubits |H〉 and |ψ1〉 (withϕ=3π/2). The system demonstrates robustness against both forms of decoherence and the CTC advantage persists up toand, respectively. The semi-transparent blue surface represents the optimum in standard quantum mechanics. Error bars obtained from a Monte Carlo routine simulating the Poissonian counting statistics are too small to be visible on the scale of this plot. Figure 6: State discrimination as a function of gate and qubit decoherence for locally prepared states. Here ε quantifies the decoherence of the unitary interaction CU xz (with θ xz = π /4), which has no analogue in the standard quantum mechanics case, and p the single-qubit depolarization of the input qubits | H 〉 and | ψ 1 〉 (with ϕ =3 π /2). The system demonstrates robustness against both forms of decoherence and the CTC advantage persists up to and , respectively. The semi-transparent blue surface represents the optimum in standard quantum mechanics. Error bars obtained from a Monte Carlo routine simulating the Poissonian counting statistics are too small to be visible on the scale of this plot. Full size image It is worth noting that the interpretation of decoherence effects in the circuit in Fig. 2a ) is very different from the linear scenario without a CTC. In the case of single-qubit depolarization the initially pure input state becomes mixed. In contrast to the linear case now an important distinction has to be made with respect to the origin of the decoherence. If it results from an interaction with the environment, which is the case considered here, then ρ CTC ‘sees’ an improper mixture and adjusts to the mixed density matrix of the input state. If, however, the origin of the mixture is classical fluctuations in the preparation apparatus, then shot-by-shot pure states enter the circuit and the consistency relation holds accordingly shot-by-shot, resulting in a proper mixture at the output. This suggests that in the presence of a CTC it would be possible to identify the origin of the decoherence in an experimental setup. Furthermore, careful analysis of the decoherence of the unitary gate CU xz reveals parallels to the effects seen in non-local state preparation. The decoherence is assumed to arise from non-local coupling to the environment. Again, due to a lack of classical knowledge of the outcome of an eventual measurement of the environment, ρ CTC ‘sees’ the mixed process in equation (7) in every run of the experiment. In the case of full decoherence the distinguishability is reduced to 0.5 as in standard quantum mechanics. The differences between local and non-local decoherence in their interpretation and effect is one of the key insights from our simulation. Quantum simulation is a versatile and powerful tool for investigating quantum systems that are hard or even impossible to access in practice [20] . Although no CTCs have been discovered to date, quantum simulation nonetheless enables us to study their unique properties and behaviour. Here we simulated the immediate adaption of ρ CTC to changes in the CTC’s environment and in particular the effect of different forms of decoherence. We also show that the nonlinearity inherent in the system is in fact not uniform (as shown in Fig. 3 ), suggesting that nonlinear effects only become apparent in certain scenarios and for a specific set of measurements. Moreover, we find intriguing differences with respect to nominally equivalent ways of pure state preparation. Although acknowledged in ref. 29 , this feature has not been further investigated in the present literature. Importantly, this effect arises due to consistency with relativity, in contrast to the similar effect for mixed quantum states discussed earlier, which is a direct result of the nonlinearity of the system [7] . Our study of the Deutsch model provides insights into the role of causal structures and nonlinearities in quantum mechanics, which is essential for an eventual reconciliation with general relativity. How to cite this article: Ringbauer, M. et al. Experimental simulation of closed timelike curves. Nat. Commun. 5:4145 doi: 10.1038/ncomms5145 (2014).